Global conservation of phylogenetic diversity captures more than just functional diversity 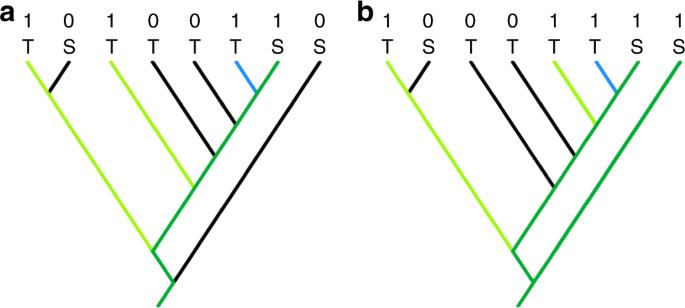Fig. 1 The disconnect between local and global PD priorities. A hypothetical phylogenetic tree of corals showing species presence/absence and PD conservation priorities in two hypothetical ecosystems:areef A,breef B. EDGE does not simply maximise PD, in contrast to Mazel et al.’s2description of the phylogenetic gambit; it uses a range of extinction probabilities for PD priority setting, which we examine here under Mazel et al.’s2focus on local-priority setting. Here, for simplicity, we maximise branch lengths, in assuming that T denotes threatened species with probability of extinction of 1 in the absence of conservation action, and S denotes secure species with probability of extinction of 0. For reefs A and B, 1 and 0 designate presence/absence of species. For each reef, dark green shows already-secure PD associated with secure species. Conservation priorities are determined under a hypothetical budget allowing selection of 2 out of the 3 threatened species (shown in light green) in order to produce a maximum gain in local secured PD. As a result, the species with the blue terminal branch is not selected for conservation in either reef. In this example, we assume that this species is only found in these two reefs; thus, such a narrow ecosystem-level priority setting approach actually allows this species, and its terminal branch, to be lost globally 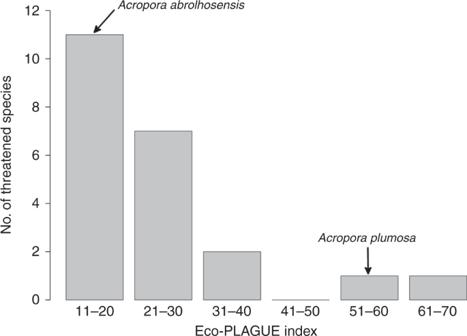Fig. 2 Local priority-setting may allow global coral PD loss. This histogram summarises the extent to which local (within-ecosystem) priority setting for 94 threatenedAcroporacorals allows possible consequent global losses. Local priority-setting explored a range of nominated budgets (for all 141 ecosystems, the budget is the number of species that can be selected for conservation in each ecosystem). For each species, we identified the minimum budget required for it to be selected in at least one ecosystem. This minimum-budget defines the Eco-PLAGUE index, reflecting how much Ecosystem Prioritizing Locally Allows Globally Unexpected Extinction. A larger Eco-PLAGUE index value indicates a greater possibility of global loss of the species, because avoiding loss requires a higher local budget to include this species as part of those selected to be conserved. Many (72) of the 94 threatened species have low (<10) Eco-PLAGUE values and thus would be selected multiple times in individual ecosystems, assuring their conservation. However, the histogram illustrates 22 species with larger Eco-PLAGUE values, showing the total number of these threatened species (y-axis) that each require a minimum local budget (Eco-PLAGUE value;x-axis) to ensure that the species is selected in at least one ecosystem, so avoiding global loss. For example,Acropora plumosahas a very large Eco-PLAGUE index of 57, meaning that it would be less likely to be selected under a local priority-setting approach, and hence more likely to be lost globally, compared toAcropora abrolhosensiswhich has a lower Eco-PLAGUE index of 16 To illustrate how localised PD priority-setting allows global PD losses, we created a hypothetical phylogeny for eight species, each designated as threatened or secure (extinction probabilities of 1 and 0, respectively), and occurring in one or both of two local ecosystems. PD-based priority-setting within each ecosystem assumed a limited conservation budget allowing selection of the two threatened species that maximise gain in secured PD. Subsequently, global PD loss was indicated by the unsecured branches arising when species were not selected in either ecosystem. We explored this problem using existing information on Acropora corals phylogeny, distribution, and conservation status [14] . The 141 reef ecoregions formed our local reef ecosystems. Securing threatened species provided PD gains, approximated by phylogenetic terminal branch lengths. Local PD priority-setting selected threatened species in order of the magnitude of these gains, up to a nominated budget number of species, applied within each ecosystem. We tabulated: (1) for each nominated budget, species that were not selected in any ecosystem; (2) the minimum budget (applied within all ecosystems) required for each species to be selected in at least one ecosystem, avoiding global loss.